Low paternal dietary folate alters the mouse sperm epigenome and is associated with negative pregnancy outcomes Epidemiological studies suggest that a father’s diet can influence offspring health. A proposed mechanism for paternal transmission of environmental information is via the sperm epigenome. The epigenome includes heritable information such as DNA methylation. We hypothesize that the dietary supply of methyl donors will alter epigenetic reprogramming in sperm. Here we feed male mice either a folate-deficient or folate-sufficient diet throughout life. Paternal folate deficiency is associated with increased birth defects in the offspring, which include craniofacial and musculoskeletal malformations. Genome-wide DNA methylation analysis and the subsequent functional analysis identify differential methylation in sperm of genes implicated in development, chronic diseases such as cancer, diabetes, autism and schizophrenia. While >300 genes are differentially expressed in offspring placenta, only two correspond to genes with differential methylation in sperm. This model suggests epigenetic transmission may involve sperm histone H3 methylation or DNA methylation and that adequate paternal dietary folate is essential for offspring health. Epigenetic information encompasses DNA methylation, non-coding RNA and modifications to histones. It serves a critical function in the regulation of gene expression and thus development and disease. From one generation to the next, the epigenome is reprogrammed in the gametes and the embryo to allow for totipotency and to prevent the transmission of epigenetic errors. However, not all regions of the epigenome are reset, permitting the transmission of epigenetic information from parents to offspring. It has been postulated that epigenetic information passed on by the gametes allows for the transmission of information on parental environmental exposures. The underlying mechanisms implicated in epigenetic inheritance are unknown, and to date there is a lack of mechanistic evidence to support epigenomic transmission via the sperm. DNA methylation is the most studied epigenetic modification and takes place at the 5-position of cytosine residues within CpG dinucleotides and is essential for the heritable silencing and regulation of many types of DNA sequences; it occurs at about 30 million sites throughout the mammalian genome [1] . DNA methylation is involved in regulating genes that are subject to parent-of-origin imprinting. These patterns of genomic methylation are acquired in the germline beginning in utero and are completed during spermatogenesis and passed to the offspring. DNA methylation is catalysed by a family of DNA (cytosine-5)-methyltransferases and cooperates with histone modifications in the regulation of gene expression and silencing. It has long been known that disease can be transmitted via the genetic layer but new modes of inheritance via the epigenome are being discovered [2] . Whereas an organism’s genotype is relatively static throughout life, the epigenome is highly dynamic and can adapt, or be altered, in response to the internal or external environment. Recent studies suggest that there are critical windows in development where the epigenome is susceptible to the introduction of epimutations through exposure to environmental factors such as toxicants or diet [3] . Very recent studies strongly suggest that paternal transmission of disease can occur via the epigenetic layer in sperm. Chronic high-fat diets fed to Sprague–Dawley rat sires induced glucose intolerance and impaired insulin secretion in their adult female offspring [4] . In humans, nutrition in males just before puberty can alter descendents survival, and predisposition to diabetes and cardiovascular disease [5] . In these prior studies, the sperm epigenome was not analysed. Dietary components serve to modulate the availability of methyl donors for methylation reactions. The B vitamins serve as coenzymes of one carbon (C 1 ) metabolism, which is a network of biochemical reactions in which a C 1 unit is received from methyl donor nutrients and used in the methylation of DNA, RNA and proteins. Thus, agents that modulate C 1 metabolism directly or indirectly affect levels of S -adenosyl methionine, the principal methyl donor for the methylation of DNA. Thus, dietary folate levels can directly influence levels of cellular DNA methylation and consequently affect gene expression [6] . Spermatogenesis consists of a carefully coordinated series of events beginning with division of spermatogonia, followed by meiosis to produce haploid spermatids, and finally the differentiation of the spermatids into mature spermatozoa. During spermatogenesis, there are epigenetic processes unlike those in the development of any other cell type, including a massive and active demethylation of the genome to allow for its sex-specific resetting by a combination of DNA methylation and histone modifications [7] . During mammalian gamete formation, some genes acquire heritable molecular imprints through epigenetic demarcation that act to either suppress or activate the expression from one parental allele in the somatic cells of offspring. These imprints are established in a sex-specific manner in the forming gametes so that the gene ‘remembers’, so to speak, its parent of origin in the offspring. If imprinting of genes is disturbed during gametogenesis, gene expression is compromised in the resulting offspring [8] . The resultant hemizygosity imposed by imprinting is believed to confer genetic vulnerability, and errors in this process are associated with diseases such as cancer, Prader–Willi syndrome and behavioural disorders [9] . Examination of DNA methylation in sperm reveals that there are unique distributions in comparison with somatic cells [10] . Infertility as a chronic disease frequently coexists with obesity, metabolic syndrome and cardiovascular disease. Infertile men have been shown to have an altered sperm epigenome including altered levels of DNA methylation, imprinted loci defects, lower pregnancy rates and a high frequency of abnormal embryos [11] . To date, there have been a handful of studies, indicating that there can be paternal transmission of subtle effects such as metabolic state to offspring. Paternal diets high in fat or low in protein can alter the metabolism in offspring and pancreatic gene expression [4] , [12] . However, there is a paucity of evidence delineating the mechanisms underlying epigenetic inheritance from a father to offspring. In clinical studies, a positive association between folate and fertility has been observed [13] and infertility is linked with a mutation in a key enzyme in folate metabolism, 5,10-methylenetetrahydrofolate reductase (MTHFR) [14] . Although folate supplementation is recommended to women before pregnancy, and food in North America has been folate fortified since 1998 (ref. 15 ), there are certain physiological states that coincide with low serum folate. Obesity and polymorphisms in folate metabolic enzymes reduce the availability of folate for methyl donation [16] , [17] . Here we hypothesize that the availability of folate will alter the levels of DNA methylation in spermatogenesis with consequences for the sperm epigenome and pregnancy outcomes. Using an inbred C57BL/6 mouse model that was exposed to low dietary folate beginning in utero and throughout life, we show that paternal diet alters sperm DNA methylation and is associated with negative reproductive outcomes including birth defects in offspring. Remarkably, the sites of the sperm epigenome bearing changes in DNA methylation are associated to genes implicated in development and chronic disease. This study is the first to show that the folate status of the father, not just the mother, may be of equal importance in determining reproductive success in terms of healthy pregnancy outcomes. Transient effects of folate deficiency on meiosis Male inbred C57BL/6 mice received throughout life either the control folate-sufficient (FS) diet (2 mg folic acid per kg) that contained the recommended amount of folate for rodents [18] , or a folate-deficient (FD) diet (0.3 mg folic acid per kg, 14.3% of the recommended amount of folate; Fig. 1a ). Dietary exposure began in utero when epigenetic patterning in germ cells begins [19] . Testis and body weights and testis histology were examined from pups at postnatal days (PND) 6, 10, 12, 14 and 18 corresponding to the appearance of spermatogenic cell types [20] . Histological examination of testis at PND 12, when meiotic cells at the leptotene stage first appear, revealed a delay in meiotic onset in FD pups ( Fig. 1b,c,d ). There were no apparent effects of diet on Sertoli ( Supplementary Fig. S1 ) and Leydig cells ( Supplementary Fig. S2 ). Body weight of male offspring was monitored as a general gauge of health and there was no reduction of body weight in FD males compared with FS males. These findings are consistent with the C57BL/6 mice model, which was on the same FD diet for 12–14 months [21] . Histological examination of adult testes revealed no detectable morphological differences between FS and FD mice ( Fig. 1f,g ). No effects of diet were observed on spermatogenesis or sperm counts ( Fig. 1e ). Diet did not alter the weights of the body, testis or epididymides ( Supplementary Table S1 ). Adult FS ( n =54) and FD ( n =49) males remained on the diets for either 2 or 4 months and were assessed for reproductive fitness by breeding trials and examination of offspring. 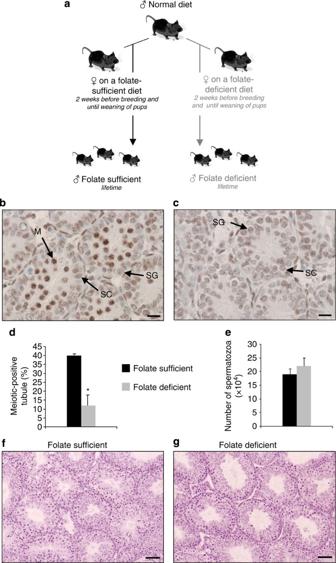Figure 1: Meiotic onset is delayed in FD mice but adult spermatogenesis is normal. (a) C57BL/6 females were fed either a FS or a FD diet, (n=64 for each) 2 weeks before breeding with a C57BL/6 male fed with control mouse chow. Females were maintained on the experimental diet through pregnancy and lactation. From weaning until throughout life, male pups received the same experimental diet as their mother. PND12 testis cross-sections from FS (b) and FD (c) testis cross-sections were stained using anti-histone H3 monomethylation at lysine 4 (H3K4-me1), a marker of early meiotic spermatocytes46. Fewer meiotic cells (M, brown staining) were present in FD tubules (c) in comparison with FS mice (b), whereas spermatogonia (SG) and sertoli cells (SC) were not affected. (d) The ratio of meiotic tubules (>10 meiotic germ cells) to total number of tubules was quantitated. Means±s.e.m. of three determinations are shown. *P<0.05 by the Mann–WhitneyU-test. Sperm counts were performed in adult FS and FD mice (e). Means±s.e.m. of five determinations are shown. *P<0.05 by Student’st-test. Spermatogenesis was assessed in adult FS (f) and FD mice (g) by haematoxilin/eosin staining. Scale bars, 10 μm (b,c) and 100 μm (d,e). Figure 1: Meiotic onset is delayed in FD mice but adult spermatogenesis is normal. ( a ) C57BL/6 females were fed either a FS or a FD diet, ( n =64 for each) 2 weeks before breeding with a C57BL/6 male fed with control mouse chow. Females were maintained on the experimental diet through pregnancy and lactation. From weaning until throughout life, male pups received the same experimental diet as their mother. PND12 testis cross-sections from FS ( b ) and FD ( c ) testis cross-sections were stained using anti-histone H3 monomethylation at lysine 4 (H3K4-me1), a marker of early meiotic spermatocytes [46] . Fewer meiotic cells (M, brown staining) were present in FD tubules ( c ) in comparison with FS mice ( b ), whereas spermatogonia (SG) and sertoli cells (SC) were not affected. ( d ) The ratio of meiotic tubules (>10 meiotic germ cells) to total number of tubules was quantitated. Means±s.e.m. of three determinations are shown. * P <0.05 by the Mann–Whitney U -test. Sperm counts were performed in adult FS and FD mice ( e ). Means±s.e.m. of five determinations are shown. * P <0.05 by Student’s t -test. Spermatogenesis was assessed in adult FS ( f ) and FD mice ( g ) by haematoxilin/eosin staining. Scale bars, 10 μm ( b , c ) and 100 μm ( d , e ). Full size image Folate deficiency increases DNA damage in spermatocytes Folate deficiency has been linked to increased DNA breaks owing to excessive uracil incorporation [22] . The most damaging DNA breaks in terms of genome integrity are DNA double-strand breaks (DSBs) [23] . Terminal deoxynucleotidyl transferase-mediated dUTP nick-end labelling immunostaining was used to detect cellular DNA fragmentation and to assess apoptosis. No spermatogenic stage-specific apoptosis was observed and the proportion of apoptotic tubules was not increased in FD males, in comparison with FS males ( P >0.05 by Student’s t -test; Supplementary Fig. S3 ). As a second assessment of DNA damage, spermatocyte-enriched cell spreads were prepared from FS and FD mice. Chromosomes were co-immunolabelled with the synaptonemal complex protein 3 (SYCP3) and the phosphorylated histone variant, γ-H2AX ( Supplementary Fig. S4 ). The γ-H2AX variant is involved in DNA repair activities and the targeting of DNA DSBs [24] . In meiotic prophase I, γ-H2AX foci are present as part of the molecular mechanisms mediating recombination. The number of γ-H2AX peaks in leptotene spermatocytes with 300 foci per cell and gradually decreases to 120 foci per cell in early pachytene, and to 48 in late pachytene [25] . Consistent with previous studies, the sex body was intensely stained by γ-H2AX ( Supplementary Fig. S4a–d ) and the number of foci observed was on average 125.5±2.1 in early pachytene and 58.5±1.9 in late pachytene of FS [25] . In early and late pachytene spermatocytes from FD mice, γ-H2AX foci were significantly increased suggesting DNA damage. As meiotic prophase progressed, the difference in the foci number between FS and FD cells increased from 5.9% in early pachytene to 12.5% in late pachytene spermatocytes ( Supplementary Fig. S4e ). To determine whether DNA damage in spermatocytes of FD mice was sustained in the sperm or was repaired, a Comet assay was carried out on sperm from FS and FD mice to measure DNA single-strand and DSBs [26] . The Comet assay revealed no differences in the DNA fragment level as represented by tail DNA, tail length and tail extent moment ( P >0.05 by Student’s t -test; Table 1 ), indicating that DNA damage in FD spermatocytes was repaired. Table 1 Assessment of sperm chromatin integrity for the folate-sufficient (FS) and deficient (FD) mice by Comet assay. Full size table Somatic cells are not affected by folate deficiency To determine whether somatic cells in the testis were sensitive to folate deficiency, we examined Sertoli and Leydig cell development at critical points following their proliferation and differentiation [27] , [28] . It is believed that the total number of Sertoli cells determines the efficiency of spermatogenesis [29] . Thus, we examined the Sertoli number at PND10 (FS, n =3; FD, n =3), since in mice Sertoli cells proliferate only in fetal/neonatal period and become almost quiescent at PND12 (ref. 27 ). Sertoli cells were identified by immunofluorescent labelling with anti-MIS (Müllerian-Inhibiting Substance) and counted in 10 round tubules per animal in FS and FD ( Supplementary Fig. S1a,b ). No difference occurred in Sertoli cell numbers between FS and FD mice ( P >0.05 by the Mann–Whitney U -test; Supplementary Fig. S1c ). Leydig cells are prominent in the interstitial space and are responsible for testosterone production [30] . In mice, the fetal Leydig cells are present and observable as round to oval shaped and are found exclusively in clusters. Leydig cells start to regress postnatally marked by the scattering of clusters and their decreasing number [28] , [31] . The histological examination of testis cross-sections stained by the Leydig cell marker, 3β-HSD (3-β-Hydroxysteroid Dehydrogenase/Δ-5-4 isomerase), revealed no detectable size or quantitative differences of fetal Leydig cell clusters between FS and FD males at PND6 ( Supplementary Fig. S2 ). Adult Leydig cells (ALD) first appear at PND10–13. The first stage of ALDs, from the initiation to PND25, is the progenitor Leydig cell (PLD) stage, which has a high proliferation rate. After this stage, ALDs only double once and then become quiescent [31] . Thus, we assessed the postnatal ALD number to determine whether ALD proliferation was affected by folate deficiency. In PND12 FS and FD mice testis, the number of PLD was quantified. PLD were identified as 3β-HSD-positive cells with slender-shaped cytoplasm and an elongated nucleus, located singly around seminiferous epithelium ( Supplementary Fig. S2a,b ). The ratio of the total number of PLDs to the number of tubules counted was calculated and compared between FS and FD mice (FS, n =3; FD, n =3; Supplementary Fig. S2c ). No observable change in morphology or number of the PLDs between FD and FS testis occurred. Folate deficiency leads to negative reproductive outcomes To determine whether paternal FD diets affected fertility and pregnancy outcomes, FS and FD males were mated to reproductively robust outbred CD-1 females that received control diets. The fertility of FD males was compromised, as demonstrated by the significantly reduced pregnancy rate of 52.38% compared with 85% for FS mice ( Supplementary Fig. S5a ). There was no difference in mating behaviour as evidenced by plug-positive females but there was an increased breeding interval in females bred to FD males. We next assessed embryo loss and development at 18.5 days post conception (dpc). Litters were sired by FS ( n =32) or FD ( n =35) males. Embryo weight and crown-rump length were not affected by paternal diet ( Supplementary Table S2 ). Preimplantation loss was not affected by diet but post-implantation loss increased in FD-sired pregnancies ( Supplementary Table S3 ). This increased loss was reflected in the twofold greater resorption rate in pregnancies sired by FD males in comparison with those sired by FS males ( Supplementary Fig. S5b ). Developmental abnormalities were observed with a greater frequency in fetuses sired by FD males ( Fig. 2 ; Supplementary Table S2 and Supplementary Fig. S6 ). Of FD-sired fetuses, 27% had visible gross anatomical abnormalities versus 3% in litters sired by FS fathers ( Supplementary Table S2 ). Malformations observed in FD-sired offspring included craniofacial abnormalities such as hydrocephalus ( Fig. 2b ). Limb defects included underdeveloped digits, or in some cases anonychia and/or hind limb hyperextension ( Fig. 2c ). In several FD-sired fetuses, abnormalities included muscle and/or skeletal defects in the region of the spine or scapula ( Fig. 2d,e ). These were confirmed by histopathological analysis that revealed muscular dysplasia adjacent to the scapula ( Fig. 2f,g ). Given that the observed gross malformations indicated probable skeletal malformations, selected FS and FD fetuses were processed for skeletal analysis ( Fig. 2h–l ). Skeletal analysis confirmed abnormalities such as reduced ossification of the skull as well as a delay in the development of the digits in FD-sired offspring ( Fig. 2h,i ). In addition, misalignment or even incomplete development of the sternebrae plates was often observed in FD-sired offspring ( Fig. 2j–l ). Abnormalities observed in FS-sired offspring were minor and included a runt and skin discolouration. 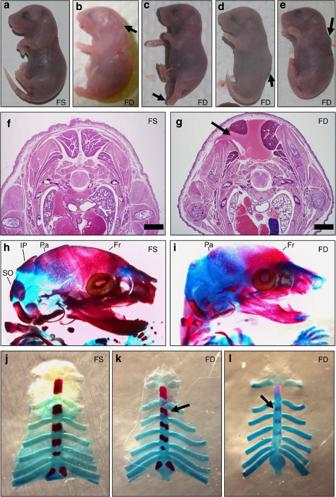Figure 2: Paternal folate deficiency increases birth defects in offspring. Fetuses sired by FD males displayed increased developmental abnormalities indicated by arrows (b–e) than those sired by FS males (a). Shown are the following: (b) hydrocephalus and associated craniofacial defects, (c) limb hyperextension with dysgenesis of digits, (d) spine malformation and (e) dorsal malformations. Histopathological analysis was carried out on selected FS- (f) and FD- (g) sired fetuses. (g) In this thoracic transverse section of an FD-sired fetus, the arrow indicates an imbalance between the right and left side muscular and bone tissues indicated muscular dysplasia. Scale bars, 1 mm (f,g). Skeletal staining was performed in both FS- (h,j) and FD- (i,k,l) sired fetuses. Bone is stained purple and cartilage blue. (i) FD-sired fetus lacking interparietal (IP) and supraoccipital (SO) bones and had underdeveloped frontal (Fr), parietal (Pr) bones and digits. FD-sired fetuses, with misaligned (k), or incomplete development (l) of the sternebrae plates. Figure 2: Paternal folate deficiency increases birth defects in offspring. Fetuses sired by FD males displayed increased developmental abnormalities indicated by arrows ( b – e ) than those sired by FS males ( a ). Shown are the following: ( b ) hydrocephalus and associated craniofacial defects, ( c ) limb hyperextension with dysgenesis of digits, ( d ) spine malformation and ( e ) dorsal malformations. Histopathological analysis was carried out on selected FS- ( f ) and FD- ( g ) sired fetuses. ( g ) In this thoracic transverse section of an FD-sired fetus, the arrow indicates an imbalance between the right and left side muscular and bone tissues indicated muscular dysplasia. Scale bars, 1 mm ( f , g ). Skeletal staining was performed in both FS- ( h , j ) and FD- ( i , k , l ) sired fetuses. Bone is stained purple and cartilage blue. ( i ) FD-sired fetus lacking interparietal (IP) and supraoccipital (SO) bones and had underdeveloped frontal (Fr), parietal (Pr) bones and digits. FD-sired fetuses, with misaligned ( k ), or incomplete development ( l ) of the sternebrae plates. Full size image Abnormalities in FD pregnancies were also detected at the level of the placenta. Development of the placenta in part depends on epigenetic information for genomic imprinting from the father [32] . While placenta weight and size did not differ between the FS and FD offspring ( Supplementary Table S2 ), there were two occurrences of fused placentas in pregnancies sired by FD fathers ( Supplementary Fig. S6a ). The embryos sharing the placenta were separately connected, but in both cases one embryo was smaller in size indicating that its development was compromised by the placental abnormality. Histopathology confirmed placenta abnormalities at the cellular level where there was an absence of the giant cell layer and an abnormally thin spongiotrophoblast layer in a pregnancy sired by a FD male ( Supplementary Fig. S6b,c ). A FD diet alters the sperm epigenome The sperm epigenome at the level of DNA methylation was assessed to determine whether folate availability altered the sperm epigenome, and whether there were epigenetic alterations at genes implicated in development and disease that correlated with the abnormal phenotypes observed in FD-sired offspring examined. Genome-wide DNA methylation was assessed by methylated DNA immunoprecipitation (MeDIP) followed by hybridization using the NimbleGen mouse 2.1 deluxe promoter array (MeDIP-chip). The sperm cells were isolated using a swim up method, which prevents contamination by somatic cells. As further validation of the purity of the sperm population, and to validate the MeDIP procedure, we assessed enrichment following DNA methylation selection by MeDIP followed by real-time PCR. Regions selected for analysis were known to be fully methylated, or not, in spermatozoa ( Supplementary Fig. S7 ). Gene regions targeted included the following: first, the imprinting control region of H19 , the paternally imprinted gene that is hypermethylated in sperm [33] , second, the promoter region of Nanog [34] also hypermethylated in sperm and, third, the promoter regions of the testis-specific variants of histones H1 ( H1t ) and H2b ( TsH2b ), which are hypomethylated in sperm and hypermethylated in somatic tissues [35] . We observed, before and after amplification with a WGA2 kit, a strong enrichment in the MeDIP fraction of H19ICR and Nanog, whereas H1t and tsH2b displayed very low signals. These results validate the purity of the sperm population and the specificity of the MeDIP before and after the amplification process. By this MeDIP-chip analysis under highly stringent criteria (false discovery rate (FDR) threshold of 0.1), 57 genomic regions had altered methylation profiles in sperm from FD males in comparison with sperm from FS ( Supplementary Table S4 ). Within these regions, methylation differences ranged from −1.33 to 2.76 (log2 fold-difference). Forty-six of these regions were located within 10 kb of the transcription start site and 31 within 5 kb. The regions beyond 10 kb were included in our analysis, as the existence of a long distance enhancer or silencer regulated by DNA methylation has been shown to influence gene expression as far as 100 kb from the gene [36] . Indeed, the methylation level of the differentially methylated region located in H19 promoter at more than 70 kb from Igf2 regulates its expression [37] . Some gene promoter regions had multiple, dispersed sites of differential methylation such as the promoter of the microRNA Mir715 ( Fig. 3a ). Other promoter regions of genes such as Ddx58 and Sfi1 had localized methylation changes close to the transcription start site ( Fig. 3b,c ). Interestingly, the methylation levels were decreased in the FD fraction for certain genes ( Fig. 3a,c ) but for others it was increased ( Fig. 3b ). At an FDR threshold of 0.25, a further 200 additional differentially methylated regions were identified and these regions were included in functional analysis using gene sets obtained from GO (Gene Ontology project), KEGG (Kyoto Encyclopedia of Genes and Genomes) and mSigDB (Molecular Signature Database), and the software DAVID (Database for Annotation Visualization and Integrated discovery) [38] . Highlights of this analysis revealed methylation differences induced by the FD diet in promoter regions located in genes implicated in development and with functions in the central nervous system, kidney, spleen, digestive tract and muscle tissue ( Table 2 ). 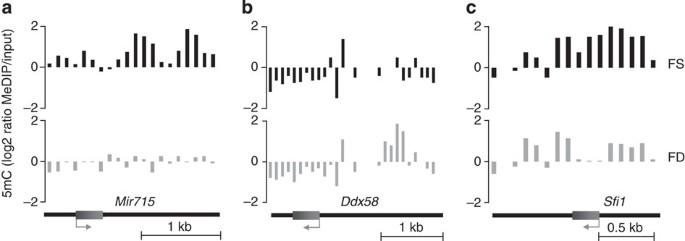Figure 3: Folate deficiency alters sperm DNA methylation. Changes in DNA methylation are illustrated by smoothed MeDIP over input log2 ratios of individual oligonucleotides for the folate-sufficient (FS) and the folate-deficient (FD) animals. The gene is indicated at the bottom of the graph and the arrow represents the transcription start site (TSS). In addition, the low-folate diet also affected the methylation status of genes associated with chronic diseases such as diabetes, autoimmune diseases, neurological diseases, autism, schizophrenia and cancer ( Table 3 ). Figure 3: Folate deficiency alters sperm DNA methylation. Changes in DNA methylation are illustrated by smoothed MeDIP over input log2 ratios of individual oligonucleotides for the folate-sufficient (FS) and the folate-deficient (FD) animals. The gene is indicated at the bottom of the graph and the arrow represents the transcription start site (TSS). Full size image Table 2 Genes implicated in development were differentially methylated in sperm of folate-deficient (FD) males compared with the folate-sufficient (FS) males. Full size table Table 3 Sperm from folate-deficient males had differential methylation in comparison with folate-sufficient males at sites associated with cancer and chronic human diseases. Full size table Less than 1% of the genome comprises imprinted genes that are also subject to epigenetic reprogramming in spermatogenesis and required for normal development of the embryo [39] . Imprinted genes have been suggested to be sensitive to environmental programming; however, none of the 65 imprinted genes tiled on the promoter array displayed any significant change in their DNA methylation profile. Selected targets were analysed by Sequenom MassARRAY, a technique based on bisulfite conversion with a resolution at the CpG level. Criteria for the selection of gene targets for validation were based on the following: first, on variation in methylation profile to confirm sensitivity over a range of methylation states (low overall methylation, or intermediate methylation or high overall methylation), which were detected by the MeDIP-array as being differentially methylated at the FDR<0.25; second, the gene had a biological link with developmental processes that corresponded to developmental abnormalities observed in offspring sired by FD males (see Fig. 2 ); third, the gene had a suitable number of CpGs for validation by the highly sensitive (single CpG resolution), and quantitative method, Sequenom MassARRAY. The genes selected for validation were the following: Rfwd2 (a ubiquitin-protein ligase expressed in the heart, testis, stomach and muscle), Sfi1 (cell signalling, widespread tissue distribution including the axial skeleton and muscle), Kdm3b (a chromatin modifier with widespread expression during embryo development), Gm52 (required for placental development) and Rbks (metabolism and cell signalling with widespread tissue distribution; Fig. 4 ). Sequenom MassArray analysis confirmed significantly altered DNA methylation at specific CpG locations for selected genes, thereby validating analysis by MeDIP-Array. 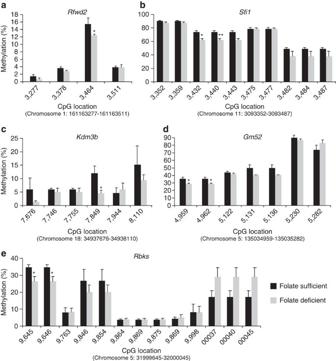Figure 4: Folate deficiency alters sperm DNA methylation at genes implicated in development and metabolic processes. Sequenom MassARRAY methylation analysis was performed on selected targets of interest identified by MeDIP-chip as altered in FD versus FS sperm. FD sperm had significantly reduced 5-methylcytosine at CpG locations ofRfwd2(a),Sfi1(b),Kdm3b(c), Gm52(d) andRbks(e). Means±s.e.m. of five determinations are shown. *P<0.05 by Student’st-test. Figure 4: Folate deficiency alters sperm DNA methylation at genes implicated in development and metabolic processes. Sequenom MassARRAY methylation analysis was performed on selected targets of interest identified by MeDIP-chip as altered in FD versus FS sperm. FD sperm had significantly reduced 5-methylcytosine at CpG locations of Rfwd2 ( a ), Sfi1 ( b ), Kdm3b ( c ) , Gm52 ( d ) and Rbks ( e ). Means±s.e.m. of five determinations are shown. * P <0.05 by Student’s t -test. Full size image Histone modifications such as histone H3 lysine 4 (H3K4) and lysine 9 (H3K9) methylation have been shown to differentially mark genes in human and mouse sperm [40] , [41] , [42] . We investigated whether folate availability could alter the sperm histone modification pattern by measuring global levels of methylation of histone H3 at K9 and K4 in epididymal sperm extracts. Sperm from FD males had significantly reduced H3K4 and K9 monomethylation compared with FS sperm, and reduced H3K9 trimethylation compared with FS sperm ( P <0.06 by Student’s t -test; Supplementary Fig. S8 ). Thus, histone methylation levels in sperm are sensitive to folate availability, and different histone methyltransferases may possess different sensitivities to an altered methyl donor pool. Altered gene expression in placenta of FD-sired offspring To determine whether there was transmission of epigenetic effects from sires to offspring, global gene expression levels were assessed in placenta from 18.5 dpc fetuses sired by either a FS or FD male ( Fig. 5 ). Analysis of array data revealed differential expression of 380 genes placenta from FD-sired offspring versus FS-sired offspring. The top 39 gene candidates selected based on their P -value are shown in Fig. 5a . Functional analysis identified 21 of those genes as implicated in the regulation of gene transduction/cell signalling. Of these differentially expressed genes, 10 were selected for validation by real-time PCR in independent samples (FS=8 placentas, FD=8 placentas each from different litters; Fig. 5b,c ). Notably, two validated genes with differential expression ( Cav1 , a cell cycle regulator, and Txndc16, a gene highly expressed in placenta with a function in cell homoeostasis) were also differentially methylated in sperm from FD males ( Supplementary Table S4 ). To determine whether the differential DNA methylation observed in FD sperm at regions near Cav1 and Txndc16 were conserved in placenta, methylation levels were measured by pyrosequencing after bisulfite conversion ( Fig. 6 ). No differences were observed between the FS- and FD-sired fetuses’ placentas at those regions. 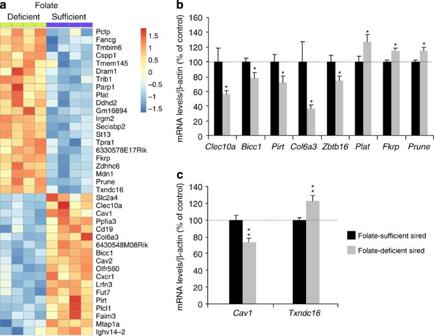Figure 5: Differential gene expression in placenta of offspring sired by FD versus FS males. (a) Heat-map showing the expression levels of 39 genes in four placentas of 18.5 dpc fetuses sired by either an FS (n=4) or FD (n=4) male. Placentas analysed were from unique litters. (b) Validation of array results by real-time PCR on an extended group of samples (n=8, FS andn=8, FD). (c) Selected array targetsCav1andTxndc16showed altered gene expression and were differentially methylated in sperm of FD sires. Data are expressed as a percentage of the control β-actin, with the value of the FS at 100%. Means±s.e.m. of eight determinations are shown. Forbandc, *P<0.05, **P<0.01 by Student’st-test. Figure 5: Differential gene expression in placenta of offspring sired by FD versus FS males. ( a ) Heat-map showing the expression levels of 39 genes in four placentas of 18.5 dpc fetuses sired by either an FS ( n =4) or FD ( n =4) male. Placentas analysed were from unique litters. ( b ) Validation of array results by real-time PCR on an extended group of samples ( n =8, FS and n =8, FD). ( c ) Selected array targets Cav1 and Txndc16 showed altered gene expression and were differentially methylated in sperm of FD sires. Data are expressed as a percentage of the control β-actin, with the value of the FS at 100%. Means±s.e.m. of eight determinations are shown. For b and c , * P <0.05, ** P <0.01 by Student’s t -test. 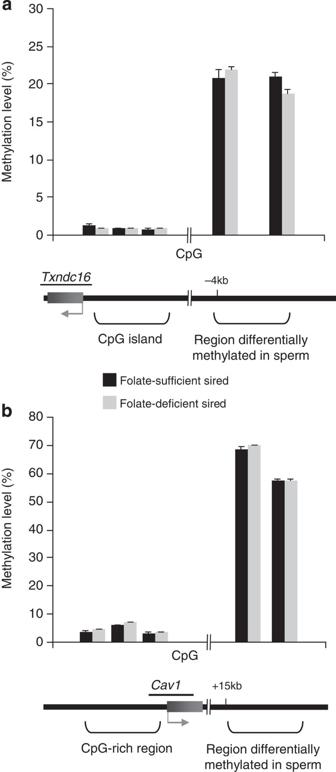Figure 6: Genomic regions located nearTxndc16andCav1that are differentially methylated in FD sperm are not differentially methylated in 18.5 dpc placentas. Pyrosequencing analysis after bisulfite conversion was carried out on 18.5 dpc placentas sired by FS and FD males (FS sired,n=4; FD sired,n=4). The values are means ±s.e.m. Full size image Figure 6: Genomic regions located near Txndc16 and Cav1 that are differentially methylated in FD sperm are not differentially methylated in 18.5 dpc placentas. Pyrosequencing analysis after bisulfite conversion was carried out on 18.5 dpc placentas sired by FS and FD males (FS sired, n =4; FD sired, n =4). The values are means ±s.e.m. Full size image In this study, we identify multiple regions of the sperm epigenome that are environmentally programmed by factors in the diet. There are three major epigenomic reprogramming periods in the lifetime of male mammals. This massive resetting is essential to allow for the germ cell-specific epigenetic programme to be established, which is required for embryo totipotency and for the removal of epigenetic mutations to prevent the transmission of disease. In the preimplantation embryo, the epigenome is reprogrammed when DNA methylation and histone methylation are actively removed with the exception of imprinted genes, repeat sequences and unidentified regions that are involved in the epigenetic inheritance of disease [43] , [44] . Epigenetic marks are then re-acquired in a sex-, cell- and tissue-specific manner in the peri-implantation period. The second period of reprogramming also takes place in utero and the target is the primordial germ cells within the developing embryo. As two major periods of epigenomic programming occur in utero, this emphasizes that this is a critical window in life for the induction of epigenetic defects. The results of this study highlight the importance of the in utero environment and show that dietary exposures in utero affected the health of two generations: the fathers’ reproductive health (F1) and the offspring (F2). The third period of epigenomic reprogramming coincides with the onset of spermatogenesis and spans from puberty to adulthood. It is estimated that 1,000 spermatozoa are produced with every heart beat [45] , and beginning with the stem cell suppliers up to the mature sperm there are ongoing epigenomic programmes that could be influenced by the environment. It remains to be determined how sensitive epigenome reprogramming is in spermatogenesis in the adults. The results of this study lend further support to the notion that epigenetic marks in spermatogenesis are dynamic and flexible; thus, they can be modified by nutritional, hormonal and toxin exposures [46] . In this study, we demonstrate that a father’s FD diet altered the sperm epigenome and that these changes were associated to genes implicated in development and chronic disease. The functional analysis of the altered sperm methylome suggests that these offspring may be at increased risk for later chronic diseases such as diabetes and cancer. The FD model is relevant in today’s society despite folate supplementation of food. In humans, obesity and its metabolic sequelae are known to alter folate metabolism [17] . In overweight and obese individuals, homocysteine is consistently elevated [47] , whereas there are conflicting reports of effects on vitamin B12 and folate. In some studies, obesity has been associated with reduced B12 and folic acid and increased plasma homocysteine [48] , whereas others have reported only increased plasma homocysteine [14] , [47] . Differences may be due in part to ethnicity and genetic variation in folate metabolism [49] . Folate and homocysteine levels can modulate the availability of S -adenosyl methionine, the principal methyl donor. In cases of low folate or high homocysteine, methyl donor levels are reduced and can directly influence methylation of DNA [3] . In line with our dietary exposure beginning in utero is that obesity in pregnancy has been associated with lower serum folate [50] . However, it is not just the poor diet, obese and overweight populations to which our model applies. Folate metabolism depends on gene variation, obesity and diet. It is directly involved in immediate health effects such as reduced fertility and chronic disease [51] , [52] . MTHFR plays a central role in folate metabolism irreversibly converting 5,10-methylenetetrahydrofolate to 5-methylenetetrahydrofolate, the primary circulating form of folate that provides methyl groups for synthesis of methionine. A decreased pool of methyl groups will affect DNA methylation. The gene encoding 5,10-MTHFR, is located at 1p36.3 (refs 49 , 53 ). An estimated 5–20% of males are expected to have the most common polymorphisms in MTHFR and folate status can be perturbed by polymorphisms in these genes. Importantly, MTHFR is most highly expressed in the testes where there are massive changes in the levels of DNA methylation associated with sperm development and epigenetic reprogramming [54] . Indeed, mice null for Mthfr are infertile [55] . The MTHFR C677T variant has been implicated in increased risks for disease and poor outcomes for chronic disease, reproduction and cancer. Deficiencies in folate metabolism or altered homocysteine status will cause changes in gene regulation via alterations to the epigenome. Results presented here indicate that in the male there are downstream consequences for reproductive success and offspring health. Here we report that folate deficiency is associated with altered sperm DNA methylation of genes such as Aff3 , Nkx2-2 and Uts2 , which are implicated in diabetes. Our data suggest that the metabolic status of a father in terms of folate availability differentially marks sperm for DNA methylation. Does this then predispose his offspring to metabolic conditions? The increasing rates of diabetes in the USA from 6 million in 1985 to more than 20 million in 2010 indicate that the role of the sperm epigenome in this phenomena and other chronic disease warrants deeper investigation. Birth defects are the leading cause of infant mortality and developmental disabilities in the United States. Current rates of birth defects in Western society are 3%; however, the causes of 43% of those remain unknown [56] . It is well established that exposure in utero to different lifestyle factors such as diet, drugs or alcohol can alter embryo development. For instance, the role of folate deficiency of the pregnant mother in neural tube defects has long been known [57] . However, no studies have investigated the role of paternal folate status and birth defects in offspring. Here we demonstrate that defects in offspring are associated with folate deficiency in the father. Previous studies have linked sperm DNA damage to increased pregnancy loss and embryo malformations [58] , [59] . To determine whether increased embryo loss in the FD-sired pregnancies could be attributable to increased DNA damage, we assessed DNA breaks in spermatogenesis and sperm. Although there was an increased incidence of DSBs as assess by γ-H2AX foci, spermatocytes, sperm was found to be free of DNA damage as assessed by Comet assay. Thus, we suggest that the developmental abnormalities and increased pregnancy loss in FD-sired pregnancies may be attributable to the altered sperm epigenome. The wide range of abnormalities observed in offspring correlated with DNA methylation changes in sperm at a significant number of genes implicated in development. These included genes such as Lhx6 and Ets1 , which function in the development of the central nervous system, Tcf21 in kidney development and Prox1 , which regulates muscle development. There is a paucity of information showing epigenetic transmission through the germline. While our study indicates that epigenetic transmission is a possibility, overlap between genes that were identified as being differentially methylated in sperm and differentially expressed in placenta was limited to two genes. Moreover, these genes did not show methylation differences in the placenta. The development of the placenta and embryo is one of rapid cell division and differentiation. Thus, the changes in the sperm that might be reflected in the embryonic tissues may only be present for a particular window of development making them difficult to detect. Another possibility is that mechanisms other than DNA methylation are involved such as other chromatin modifiers. Notably, histone methylation in sperm was also altered by folate deficiency, and histone methylation has been localized to genes implicated in development [42] , [60] . These observations indicate that the male preconception diet and overall health status may be of equal importance as the mother’s and that the sperm epigenome plays a key role in the development of the embryo as has been suggested by recent studies [41] , [42] . Importantly, this study indicates that there are environment sensitive regions of the sperm epigenome that respond to diet and transfer a so-called epigenomic map that influences development, and perhaps in the long-term metabolism and disease in offspring. This information opens new avenues of understanding and preventing paternal routes to developmental defects and the potential mechanisms underlying inter-generational disease transmission. Animals and dietary treatments To minimize genetic noise, the inbred C57BL/6 strain was used for generation of experimental males and for analysis of the sperm epigenome. Breeding assessment of experimental males was done with the outbred CD-1 strain (Charles River Laboratories, St-Constant, QC, Canada). Mice were housed under a controlled light/dark cycle and were provided with food and water ad libitum . All animal procedures were approved by the Animal Care and Use Committee of McGill University, Montreal. Dietary exposures began in utero . To generate experimental males, female C57BL/6 were fed either the FS (2 mg folic acid per kg, n =69) diet (TD.01369, Harlan Laboratories, Madison, WI) or the FD diet (0.3 mg folic acid per kg, n =64; TD.01546), 2 weeks before breeding with non-experimental C57BL/6 males that were fed regular mouse chow (8640 Rodent diet; used only for breeding to generate experimental males; Fig. 1 ). The effects of these diets on serum levels of folate and homocysteine have been fully described in different mouse strains [21] , [61] . To breed C57BL/6 females, C57BL/6 males were brought to the females’ cages at night and removed in the morning to limit consumption of the experimental diets by the males. Females were maintained on the experimental diets through pregnancy and lactation. From weaning at PND21, male pups were given the same experimental diet as their in utero exposure until killing as adults. Antibodies Primary antibodies used in this study were anti-H3K4-me1 (ab8895, Abcam, 1:1000), anti-H3K9-me1 (ab8896, 1:1000), anti-H3K9me3 (07-442, Millipore, 1:1000), anti-β-actin (A-1978, Sigma), anti-SYCP3 (ab15093; 1:100), anti-γH2AX (05-636; 1:100), anti-MIS (sc-6886, Santa Cruz; 1:50), anti-mouse VASA homologue (in house, 1:200), anti-3βHSD (sc-30820, 1:100) and anti-5-methylcytidine (BI-MECY-0100, Eurogentec, 10 μg per immunoprecipitation tube). Secondary antibodies were horseradish peroxidase (HRP)-conjugated donkey-anti-rabbit and anti-mouse antibodies (711-035-152 and 715-035-150, Jackson Immunoresearch Laboratories, 1:500 for immunohistochemistry and 1:5000 for western blotting), Alexa Fluor 488 goat-anti-mouse (A11001, Invitrogen, 1:1000) and Alexa Fluor 594 goat-anti-rabbit (A11012, 1:1000). Immunostaining Tissues were fixed in Bouin’s or 4% buffered formaldehyde solution, processed for embedding in paraffin, and sectioned using standard histological protocols. Immunohistochemical staining was performed on 5-μm-thick sections. Tissues were then deparaffinized and rehydrated. After washing in PBS with 0.05% Brij for immunohistochemistry or PBS with 0.03% TritonX for immunofluorescence for 10 min, antigen retrieval was performed by incubating tissue sections in sodium citrate buffer (pH 6.0), heating in the microwave until boiling, followed by cooling for 30 min at room temperature. The slides were then rinsed in PBS solution and endogenous peroxidase activity was blocked by incubation with 0.3% hydrogen peroxide in methanol for 30 min at room temperature only for immunohistochemistry. The sections were subsequently blocked in 5% BSA in PBS solution for 1 h, and then incubated with the corresponding primary antibody with rocking overnight at 4 °C. After washing, the sections were incubated with secondary HRP-conjugated or fluorescence-conjugated antibody for 1 h at room temperature, followed by washing. For immunohistochemistry, immune complexes were revealed by diaminobenzidine (Sigma) and sections were counterstained with haematoxylin. For immunofluorescence, sections were mounted in Vectashield (H1200, Vector) containing 4′,6-diamidino-2-phenylindole. Reactivity was viewed using a Nikon eclipse 80i microscope (Nikon, Mississauga, Canada). Homogenization-resistant sperm counts The two caput epididymides were used for each animal at 15 weeks (FS, n =5; FD, n =5). Tissues were thawed on ice in a solution containing 0.5% Triton X-100 and then homogenized using a tissue homogenizer. Finally, sperm heads were counted using a haemocytometer. Cell preparation for analysis of DNA DSBs DNA DSBs were assessed in enriched pachytene spermatocyte cell spreads. Cells were prepared according to the drying-down technique described by Peters et al. [62] . Tubules were removed from testes and placed in hypotonic extraction buffer (30 mM Tris–HCl, 50 mM sucrose, 17 mM trisodium citrate dihydrate, 5 mM EDTA, 0.5 mM dithiothreitol and proteinase inhibitor cocktail; pH 8.2) for 60 min. Subsequently, tubules were minced into a cloudy suspension in a sucrose solution (100 mM; pH 8.2), which was then dispersed on slides pre-dipped in 1% paraformaldehyde. The slides were washed in 0.4% Photoflo (Kodak) solution and dried. Co-immunofluorescent staining of SYCP3 and γ-H2AX was then performed. Reactivity was visualized using a confocal microscope Zeiss LSM 510–NLO. Assessing DNA integrity in sperm using the COMET assay DNA single- and DSBs in spermatozoa of adult male mice were evaluated by the alkaline COMET assay [63] . Briefly, epididymal sperms were collected from 18-week-old FS and FD mice (both n =3). Fifty microlitres of sperm suspension was mixed with 500 μl 0.7% molten low-melting point agarose at 42 °C. Fifty microlitres was immediately pipetted and evenly spread onto slides. Cells were then lysed in lysis buffer (2.5 mol NaCl, 100 mmol EDTA, 10 mmol Tris–HCl, 10% dimethyl sulfoxide, 1% Triton X-100 and 40 mmol dithiothreitol; pH 10) for 1 h at 4 °C. After washing, slides were incubated in an alkaline solution (1 mmol EDTA; pH 12.3) for 45 min at 4 °C. Slides were then washed in 1 × TAE buffer for 5 min before electrophoresis at 0.7 V cm −1 for 10 min. Finally, the slides were dehydrated with 70% ethanol. DNA was stained by 1:10,000 SYBR Green (Trevigen) and pictures were immediately captured under microscope. For each animal, 100 cells were randomly selected and measured using the KOMET 5.0 image analysis system (Kinetic Imaging Ltd, Liverpool, UK). Detection of apoptotic germ cells Germ cell apoptosis was examined in testis cross-sections from 15-week-old mice using the terminal deoxynucleotidyl transferase-mediated dUTP nick-end labelling detection protocol (Apoptag, Chemicon International). All the tubules in each testis section were counted and the ratio of tubules with a certain level of apoptotic cells (>5, >10 or >15) to total number of tubules counted were calculated. Breeding trial The effect of folate deficiency on male fertility was examined by mating each experimental male (FS, n =20; FD, n =21; 8–10 weeks old) to a virgin CD-1 female over a 5-day period. Females were examined daily for vaginal plugs. Pregnancy rate was determined as the percentage of plug-positive females that became pregnant. Examination of fetuses and placentas To determine whether the offspring health was sensitive to paternal diet, CD-1 mice were mated to males fed either the FS or FD diet throughout life (FS, n =32; FD, n =35; 2–3 months old) and pregnancy outcomes were determined at 18.5 dpc. Females were killed and the number of corpora lutea (CL) on the ovary was counted. The uteri were opened and the number of resorption sites, implantation sites and live fetuses was determined. Preimplantation loss was calculated as (CL−number of implants)/CL × 100 (ref. 64 ). Post-implantation loss was calculated as (number of implants−viable fetuses)/number of implants × 100. Skeletal preparation and histopathology Alcian blue and Alizarin red staining of cleared skeletal preparations was performed according to Hogan et al. [65] . Fetuses (18.5 dpc) were fixed in 80% ethanol for 48 h. The skin and viscera were then removed and the fetuses were further fixed in 95% ethanol overnight and stained with an alcian blue solution for 12 h. After washes in 95% ethanol for 5 h, the fetuses were transferred in a 2% KOH solution for 24 h after which the muscles were removed. The remaining bones and cartilages were stained in a 1% KOH with 0.015% alizarin red S solution for 12 h, washed for 2 days in a 1% KOH with 20% glycerol solution and finally stored in glycerol. For histopathology, specimens were fixed in Bouin’s fluid and embedded in paraffin. Deparaffinized sections were stained with haematoxylin and eosin and analysed by McGill University Comparative Pathology Services. Methylation profiling by MeDIP-array The MeDIP assay was performed as described by Weber et al. [66] on sperm from FS males ( n =3) and FD males ( n =4 animals). Genomic DNA was extracted with a DNeasy Mini Kit (Qiagen, Mississauga, Canada). This DNA was then sonicated (Misonix) to obtain fragments between 300 and 500 bp. Then, 4 μg of this sonicated genomic DNA was denatured for 10 min at 95 °C and immunoprecipitated for 2 h at 4 °C with an anti 5-methylcytidine. Then, dynabeads coupled with a sheep anti-mouse-IgG antibody (Dynal Biotech) for 2 h at 4 °C were added to the mixture. After washing, proteinase K was added to the beads–DNA complex for 3 h at 50 °C and the methylated DNA was isolated by phenolchloroform extraction followed by ethanol precipitation. Input samples were processed in parallel. Immunoprecipitated DNA and input DNA from MeDIP were amplified with the GenomePlex Complete Whole Genome Amplification Kit (Sigma, WGA2) according to the manufacturer’s instructions. Array hybridization using the NimbleGen mouse 2.1 deluxe promoter array was then carried out by Nimblegen. Microarray analysis Microarrays were processed and probe intensities were extracted by Nimblegen. Extracted probe intensities were then analysed using the R software environment for statistical computing. Log ratios of the bound (Cy5) and input (Cy3) microarray channel intensities were computed for each microarray, and then microarrays were normalized to one another using quantile normalization [67] under the assumption that all samples have identical overall methylation levels. The resulting values for each probe are called normalized intensities. Differential methylation between groups of samples was determined in two stages to ensure both statistical significance and biological relevance. In the first stage, normalized probe intensity differences between FD and FS microarrays were obtained for each probe (FD–FS). Given that the DNA samples were sonicated before hybridization, we assumed that probes within 500 bp should approximately agree. Genomic regions tiled with probes were partitioned into 1,000 bp regions, each containing ~10 probes. For each such 1,000 bp region, we calculated the significance of enrichment for high or low normalized probe differences of probes within its promoter. Significance was determined using the Wilcoxon rank-sum test comparing differences of these probes against those of all the probes on the microarray. The resulting P -values for each gene were then corrected for multiple testing by calculating their FDR using the Benjamini and Hochberg algorithm. A probe was then called differentially methylated if it satisfied each of the following: the region containing it had a FDR of at most 0.1 and the normalized intensity difference between FD and FS for the probe was greater than 1 or less than −1. The methylation level of a probe or site, when estimated from microarray data, was obtained by applying a Bayesian deconvolution algorithm [68] to normalized probe intensities and corresponding sequence information indicating the locations of CpG dinucleotides. All functional analysis was based on gene sets obtained from GO, KEGG and mSigDB. A gene was included in this analysis if at least one probe between −8,000 bp and 2,000 bp of its transcription start was called differentially methylated. A small number of genes were initially included ( Supplementary Table S4 ); consequently, we relaxed the requirements for calling a probe differentially methylated but increasing the FDR threshold from 0.1 to 0.25. Transcription start sites for the mouse gene were obtained from BiomaRt ( http://www.biomart.org/ ). Functional significance was determined by applying the hypergeometric to the overlap between gene sets and genes called differentially methylated. Gene expression levels from mouse testes were obtained from published data [69] . These were used to partition genes by expression percentiles (0–5, 5–10,..., 95–100). To obtain gene promoter methylation levels, we computed the average normalized intensity of each probe across both microarrays and then applied the Bayesian deconvolution algorithm mentioned above to the resulting averages. Sequenom MassARRAY methylation analysis One microgram of DNA from FS ( n =5) and FD ( n =5) sperm was bisulfite treated with EZ DNA Methylation Gold Kit (Zymoresearch, D5007). Primers to amplify different amplicons in specific regions of Rfwd2 Sfi1 Kdm3b , Gm52 and Rbks were designed using the Sequenom EpiDesigner application. Sequenom MassARRAY methylation analysis was then performed using the MassARRAY Compact System (Sequenom, Inc. San Diego, CA). This system is based on mass spectrometry analysis for qualitative and quantitative detection of DNA methylation using homogeneous MassCLEAVE base-specific cleavage and matrix-assisted laser desorption/ionization time-of-flight mass spectrometry. Spectra were elaborated by the Epityper software v1.2.0 (Sequenom, Inc.), which provides methylation values of each CpG unit expressed as percentage. Those values result from the calculation of the ratio mass signals between the methylated and non-methylated DNA. Gene expression array Total RNA was extracted from the placenta from different litters from 18.5 dpc fetuses sired by either a FS male ( n =4) or a FD male ( n =4), using the RNeasy Mini Kit (Qiagen, Mississauga, Canada) according to the manufacturer’s instructions. Cyanine 3-labelled CTP complementary RNA was produced using the Low Input Quick Amp Labeling Kit, according to manufacturer’s instructions (Agilent Technologies, Mississauga, Canada). The labelled complementary RNA was then normalized, fragmented and hybridized on SurePrint G3 Mouse GE 8 × 60 K arrays. The arrays were incubated in an Agilent Hybridization oven at 65 °C for 17 h at 10 r.p.m. They were washed and scanned on an Agilent DNA Microarray Scanner C. Output from the Agilent Feature Extraction software were read into R, preprocessed and tested for differential expression using functions from the Bioconductor package Limma. The normexp method with an offset value of 16 was used for global background adjustment, followed by quantile normalization and a log2 transformation. The annotation for probes was retrieved from the Gene Expression Omnibus. Using the appropriate Limma functions, a linear model was fit to each gene separately. This linear model included the paternal diet as a categorical variable. Moderated t -tests were performed on the difference between the FD and FS paternal diet groups. False discovery rate (FDR) estimation was carried out using the Benjamini–Hochberg method. Candidates for validation were selected from a list of relaxed statistical significance, defined as genes with P <0.01 (determined by the aforementioned moderated t -tests) and a minimal absolute fold-change value of 1.2. Reverse transcription and real-time PCR Total RNA was extracted using the RNeasy Mini Kit (Qiagen) according to the manufacturer’s instructions and 1 μg of total RNA was reverse transcribed using the High Capacity cDNA Reverse Transcription kit (Applied Biosystems, Foster City, CA, USA). Primers were designed using Primer Express software (Applied Biosystems; Supplementary Table S2 ). PCR reactions were performed following the SYBR Green Universal PCR Master Mix protocol (Applied Biosystems) using an ABI Prism 7500 apparatus (Applied Biosystems). Each sample was run in triplicate and negative controls (non-template control and minus reverse transcription samples) were run for each primer pair. The measured amount of each complementary DNA was normalized using the control β-actin, a housekeeping gene with expression that was not altered by treatment. The relative quantification was performed using the standard curve method. A list of the primers used is provided in Supplementary Table S5 . Western blotting Western blots were performed to measure global levels of histone methylation in FS and FD sperm. Sperm extracts were prepared in Laemmli buffer (50 mM Tris–HCl (pH 7.5), 170 mM NaCl, 1% NP-40, 50 mM NAF, 1 mM phenylmethylsulfonyl fluoride, 100 μM NaVO 3 and a proteinase inhibitor cocktail). Equal amounts of protein were resolved by standard SDS–polyacrylamide gel electrophoresis and electroblotted onto nitrocellulose membranes. The membranes were incubated overnight at 4 °C in PBS that contained 5% low-fat milk, 0.05% Tween-20 and the corresponding first antibody. After washing, the membranes were incubated with a donkey-anti-rabbit or anti-mouse HRP-conjugated secondary antibody diluted in 5% milk in PBS with 0.05% Tween-20, and labelling was detected using enhanced chemiluminescence (Pierce). Membranes were exposed to Kodak autoradiography BioMax film. Films were scanned and the band intensity was quantified using AlphaDigiDocTM. Each experiment was performed on six FD and six FS sperm samples and replicated a minimum of three times. Full-size blots are shown in Supplementary Fig. S9 . Pyrosequencing DNA methylation levels in placenta were determined by pyrosequencing using a PyroMark Q24 (Qiagen) after bisulfite conversion, which is a real-time sequencing-based DNA analysis that quantifies multiple and consecutive CpG sites individually. Placental DNA was extracted using the DNeasy Mini Kit (Qiagen); 1 μg of DNA was then bisulfite-treated using the EpiTect Fast DNA Bisulfite Kit (Qiagen). Bisulfite-treated DNA was eluted in 15 μl volume, and 3 μl was used for each PCR. PCR was performed using the HotStar DNA Polymerase (Qiagen). The PCR was performed with one of the PCR primers biotinylated to convert the PCR product to single-stranded DNA templates. The PCR products (each 20 μl) were sequenced following the manufacturer’s instructions (Qiagen). The methylation status of each locus was analysed individually as a T/C single-nucleotide polymorphism using the PyroMark Q24 Advanced software (Qiagen). The list of primers used is listed in Supplementary Table S5 . Statistical analysis In graphs or tables, numbers represent the mean±s.e.m. of at least three independent experimental units. The level of significance for all the statistical tests used in this study was set at P <0.05 and all the tests were two tailed. Statistical analysis of pregnancy rate and resorption rate used Fisher’s exact test and χ 2 -test, respectively. The data assessing DNA methylation, mRNA levels, histone methylation, weights, sperm counts and meiotic tubule counts were analysed for differences between the control and treated group by unpaired Student’s t -test or in case of failed normality by the Mann–Whitney U -test or Kolmogorov–Smirnov test. For the fertility trial and pregnancy outcomes, all the calculation and analysis were on a per male basis. For each litter, the average of embryo weights, crown-rump lengths and placenta widths and weights were calculated, then the collection of averages for the litters sired by FS males was compared with the collection of averages for the litters sired by FD males by Student’s t -test. When analysing the COMET scores, the collection averages were compared between FS and FD males by Student’s t -test. The γ-H2Ax foci were analysed by subsample model. The animals are random effects nested in the fixed effects of folate level. Each cell analysed is a subsample unit, while the animal is the experimental unit. The dietary treatments were randomized and samples were randomly selected from experimental groups for downstream analysis including for gene expression, pathology and sperm epigenome analysis. No blinding was done. All the n indicated represent biological replicates. Data were analysed with the aid of SAS 9.2 and PASW Statistics Base 18. Accession codes: The MeDIP-array data have been deposited in the Gene Expression Omnibus (GEO) repository under accession number GSE52017 . The Gene expression array data have been deposited in the GEO repository under accession number GSE51819 . How to cite this article: Lambrot, R. et al. Low paternal dietary folate alters the mouse sperm epigenome and is associated with negative pregnancy outcomes. Nat. Commun. 4:2889 doi: 10.1038/ncomms3889 (2013).